Hydrothermal vent fields and chemosynthetic biota on the world's deepest seafloor spreading centre The Mid-Cayman spreading centre is an ultraslow-spreading ridge in the Caribbean Sea. Its extreme depth and geographic isolation from other mid-ocean ridges offer insights into the effects of pressure on hydrothermal venting, and the biogeography of vent fauna. Here we report the discovery of two hydrothermal vent fields on the Mid-Cayman spreading centre. The Von Damm Vent Field is located on the upper slopes of an oceanic core complex at a depth of 2,300 m. High-temperature venting in this off-axis setting suggests that the global incidence of vent fields may be underestimated. At a depth of 4,960 m on the Mid-Cayman spreading centre axis, the Beebe Vent Field emits copper-enriched fluids and a buoyant plume that rises 1,100 m, consistent with >400 °C venting from the world's deepest known hydrothermal system. At both sites, a new morphospecies of alvinocaridid shrimp dominates faunal assemblages, which exhibit similarities to those of Mid-Atlantic vents. Since their initial discovery more than three decades ago [1] , deep-sea hydrothermal vents have provided insights into geological processes associated with seafloor spreading [2] , the geochemical mass balance of the oceans [3] and submarine ore-body formation [4] . Their associated biological assemblages have yielded more than 500 new faunal species [5] , and advanced our knowledge of species dispersal, biogeography and evolution in the deep ocean [6] . More than 75% of the 65,000-km mid-ocean ridge system, however, remains unexplored for hydrothermal activity [7] . Recent targets for exploration include ultraslow-spreading ridges [8] , [9] , [10] , [11] , which were previously considered incapable of supporting hydrothermal activity as a result of their reduced magmatic heat budget [12] . These ridges constitute 20% of the world's seafloor spreading centres [13] . Water column signals indicative of underlying hydrothermal vents have now been detected in several locations, but so far only two vent fields have been observed directly on such ridges, on the Arctic Mid-Ocean Ridge [14] and on the south west Indian Ridge [15] . The 110 km-long Mid-Cayman spreading centre (MCSC) is an ultraslow ridge, located in the Cayman Trough of the Caribbean Sea ( Fig. 1a ), and thereby isolated by 4,000 km from the contiguous mid-ocean ridge system. The MCSC has a full-spreading rate of 15 mm per year and has been active for 49 My [16] . The spreading axis of the MCSC presently consists of two second-order segments, separated by a small non-transform offset at 18°20′N ( Fig. 1b ). The depth of the spreading axis of the MCSC ranges from 4,200 to >6,000 m, which makes it the world's deepest seafloor spreading centre [17] . As pressure of the overlying water column influences the maximum temperature at which hydrothermal fluids can vent at the seafloor [18] , hydrothermal vent fields on the axis of the MCSC could exhibit exceptionally high temperatures, producing vent fluids with unusual physical and chemical properties. 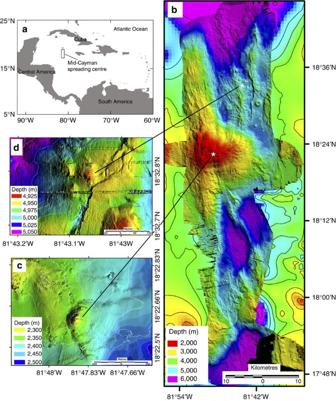Figure 1: Location of the MCSC and hydrothermal vent fields. Hydrothermal vents on the MCSC. (a) Regional location map of the MCSC. (b) Bathymetry of the MCSC, from shipboard multibeam sonar data (50-m horizontal resolution in shaded relief, against a background of GEBCO contoured bathymetry). (c) Microbathymetry of the VDVF (commemorating geochemist Karen Von Damm, 1955–2008), fromAutosub6000multibeam sonar data. (d) Microbathymetry of the BVF (named in honour of naturalist William Beebe, 1877–1962), fromAutosub6000multibeam sonar data. Figure 1: Location of the MCSC and hydrothermal vent fields. Hydrothermal vents on the MCSC. ( a ) Regional location map of the MCSC. ( b ) Bathymetry of the MCSC, from shipboard multibeam sonar data (50-m horizontal resolution in shaded relief, against a background of GEBCO contoured bathymetry). ( c ) Microbathymetry of the VDVF (commemorating geochemist Karen Von Damm, 1955–2008), from Autosub6000 multibeam sonar data. ( d ) Microbathymetry of the BVF (named in honour of naturalist William Beebe, 1877–1962), from Autosub6000 multibeam sonar data. Full size image On the western flank of the axial valley of the MCSC, there is an off-axis topographic feature known as Mount Dent, which rises 2,700 m above the spreading centre axis ( Fig. 1b ). This feature has been interpreted as an oceanic core complex (OCC) [19] , where gabbroic lower crustal and peridotite upper mantle rocks have been exposed during seafloor spreading [20] . OCCs are now recognized as common features of slow- and ultraslow-spreading ridges, and are possibly responsible for ∼ 50% of the extension along such ridges [21] . These off-axis features have been largely unexamined for high-temperature hydrothermal activity, however, because most surveys to date have focused along the spreading axes of ridges [7] . Discoveries of hydrothermal vent fields around the world have so far revealed six biogeographic provinces for vent fauna [6] , [22] , [23] , but the origin and maintenance of these provinces are poorly understood [24] , [25] . At present, the only mid-ocean ridge connection between the biogeographic provinces of the eastern Pacific and northern Mid-Atlantic occurs at high latitudes, via the Pacific-Antarctic and Indian Ocean ridge systems [6] . But before the complete closure of the Isthmus of Panama by ∼ 3.1 Ma, there was a low-latitude deep-ocean gateway between the Pacific and Atlantic via the Caribbean [26] . Chemosynthetic fauna may have dispersed across this gateway, as indicated by similarities at genus level between cold seep communities on the Oregon Margin and in the Gulf of Mexico [27] , and a high level of COI (cytochrome oxidase subunit I) gene sequence similarity among siboglinid polychaete species at cold seeps in the Gulf of Mexico and the Gulf of California [28] . Given this regional history, the MCSC was therefore identified by the international Census of Marine Life as a priority target for hydrothermal exploration, to investigate the influences of hydrography, geological history, isolation and bathymetry on global patterns of vent biogeography [6] , [25] . Water column anomalies above the MCSC consistent with underlying hydrothermal activity were reported in 2010 [11] and guided the observation, sampling and analysis of MCSC hydrothermal vent fields that we report here. We have discovered two hydrothermal vent fields in contrasting settings: a high-temperature vent field on the upper slopes of the Mount Dent OCC, and a vent field on the ridge axis at the depth of 4,960 m, which is the world's deepest known hydrothermal system. From our vent fluid geochemistry data and geological observations, we examine a possible mechanism for high-temperature venting in the off-axis OCC setting, and suggest that high-temperature vent fields may be more common than realized along slow- and ultraslow-spreading ridges. At the deep axial site, we predict vent fluid exit temperatures at or near the critical point of seawater ( ∼ 485 °C at the in situ pressure of ∼ 500 bar) [29] from our measurements of fluid and particulate geochemistry and the rise height of the buoyant hydrothermal plume. Several of the invertebrate taxa at the MCSC vent fields appear to be new species that exhibit higher-level taxonomic affinities to those present at vents the Mid-Atlantic Ridge, rather than those found at nearer cold seep environments in the Gulf of Mexico. Detection and location of vent fields During Voyage 44 of the RRS James Cook (24 March to 21 April 2010), we used a multiplatform approach to detect, locate, directly observe and sample two hydrothermal vent fields on the MCSC. Our survey with a conductivity–temperature–depth (CTD) probe showed an isothermal water column below at depth of ∼ 2,100 m over the MCSC ( Fig. 2a ). Within this water column, we detected anomalies in suspended particulates measured by a light-scattering sensor (LSS), and redox potential signals (Eh), at ∼ 200 m above the seafloor of the upper slopes of the Mount Dent OCC ( Fig. 2b ). Missions in this area by the Autosub6000 autonomous underwater vehicle then detected strong Eh signals ( Fig. 2c ) and a temperature anomaly of +0.45 °C at an altitude of 60 m above an underlying mound on the seafloor ( Fig. 1c ). Direct visual inspection by our HyBIS TV grab revealed this to be a hydrothermal vent field at a depth of 2,300 m (the Von Damm Vent Field (VDVF), 18°22.605′N 18°47.875′W; named in commemoration of hydrothermal vent geochemist Karen Von Damm, 1955–2008). 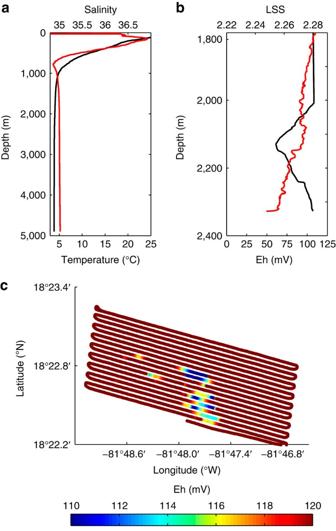Figure 2: Characteristics of the VDVF water column. (a) Profiles of temperature and salinity above the MCSC from a CTD instrument, showing a deep isothermal water column; (b) Profiles of LSS and redox potential (Eh) signals indicating the hydrothermal plume above the VDVF (c)Autosub6000survey of Eh anomalies at 60-m altitude above the VDVF. Eh values in these diagrams are the raw values of the platinum (Pt) electrode voltage against the silver–silver chloride (AgCl) reference electrode in a saturated potassium chloride (KCl) solution. Figure 2: Characteristics of the VDVF water column. ( a ) Profiles of temperature and salinity above the MCSC from a CTD instrument, showing a deep isothermal water column; ( b ) Profiles of LSS and redox potential (Eh) signals indicating the hydrothermal plume above the VDVF ( c ) Autosub6000 survey of Eh anomalies at 60-m altitude above the VDVF. Eh values in these diagrams are the raw values of the platinum (Pt) electrode voltage against the silver–silver chloride (AgCl) reference electrode in a saturated potassium chloride (KCl) solution. Full size image Our CTD survey also detected anomalies in water column particulates at an altitude of ∼ 1,100 m above the neovolcanic zone of the northern segment of the MCSC spreading centre axis ( Fig. 3a ), where a previous survey reported similar signs of underlying hydrothermal activity [11] . In addition to signals indicative of the dispersing neutrally buoyant plume from a hydrothermal vent, we encountered anomalies in particulates and Eh close to the seafloor in this area ( Fig. 3a ), consistent with the buoyant portion of that hydrothermal plume. An AUV mission at an altitude of 60 m then constrained the extent of these Eh anomalies ( Fig. 3b ), and mapped an underlying mound on the seafloor ( Fig. 1d ). Dives with the HyBIS TV grab found active hydrothermal vent chimneys on this mound, at a depth of 4,960 m (the Beebe Vent Field (BVF), 18°32.785′N 81°43.080′W; named in honour of William Beebe, 1877–1962, the first naturalist to observe deep-sea fauna in situ ). 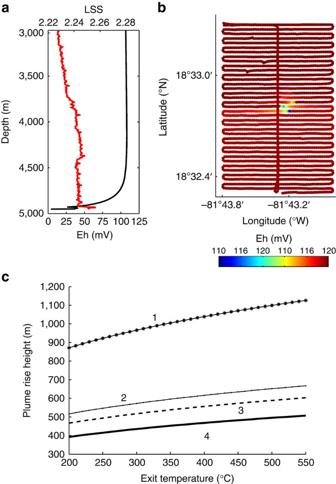Figure 3: Characteristics of the BVF water column. (a) Profiles of LSS and Eh indicating the neutrally buoyant and buoyant hydrothermal plume above the BVF. (b)Autosub6000survey of Eh anomalies at 60-m altitude above the BVF; Eh values in these diagrams are the raw values of the Pt electrode voltage against the Ag–AgCl reference electrode in a saturated KCl solution (c) Variation of plume rise height with seafloor exit temperature in the water column of the MCSC, 1, 0.2/1.5; 2, 0.1/1.5; 3, 0.2/0.5; 4, 0.1/0.5 vent area (m−2)/vertical exit velocity (ms−1), respectively, estimated from video observations at BVF. Figure 3: Characteristics of the BVF water column. ( a ) Profiles of LSS and Eh indicating the neutrally buoyant and buoyant hydrothermal plume above the BVF. ( b ) Autosub6000 survey of Eh anomalies at 60-m altitude above the BVF; Eh values in these diagrams are the raw values of the Pt electrode voltage against the Ag–AgCl reference electrode in a saturated KCl solution ( c ) Variation of plume rise height with seafloor exit temperature in the water column of the MCSC, 1, 0.2/1.5; 2, 0.1/1.5; 3, 0.2/0.5; 4, 0.1/0.5 vent area (m −2 )/vertical exit velocity (ms −1 ), respectively, estimated from video observations at BVF. Full size image The VDVF The VDVF is located on upper slopes of the Mount Dent OCC, at a distance of 13 km to the west of the neovolcanic zone that defines the active spreading axis of the MCSC. The vent field consists of a conical sulphide mound, 100 m in diameter and 30 m high ( Fig. 1c ), venting predominantly clear fluids from orifices at its peak ( Fig. 4a,b ). Samples collected by the HyBIS TV grab reveal a rubble apron of talc and serpentinite surrounding the actively venting mound. Petrographic studies reveal that the serpentinite is after a harzburgite protolith with relict orthopyroxene (now bastite) in a mesh-textured serpentinized matrix (after olivine). X-ray diffraction (XRD) analyses show talc is common and occurs with barite, gypsum and amorphous silica (quartz). Petrographic and XRD analyses of the sulphide mineral samples from the active part of the mound are predominantly composed of pyrite (iron sulphide) with some chalcopyrite (copper sulphide) and anhydrite (calcium sulphate). The presence of anhydrite indicates vent fluid temperatures in excess of 140 °C at the VDVF [30] . 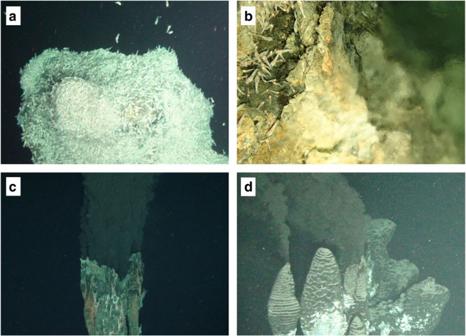Figure 4: MCSC chimneys and fauna. (a) Peak of sulphide edifice at the VDVF, depth 2,300 m, covered by an aggregation of alvinocaridid shrimp. (b) Clear vent fluids and alvinocaridid shrimp at the VDVF. (c) High-temperature venting at the BVF, depth 4,960 m. (d) Diffuser structures ornamenting sulphide chimneys at the BVF. Figure 4: MCSC chimneys and fauna. ( a ) Peak of sulphide edifice at the VDVF, depth 2,300 m, covered by an aggregation of alvinocaridid shrimp. ( b ) Clear vent fluids and alvinocaridid shrimp at the VDVF. ( c ) High-temperature venting at the BVF, depth 4,960 m. ( d ) Diffuser structures ornamenting sulphide chimneys at the BVF. Full size image We collected samples of buoyant vent fluids from an altitude of <5 m above the active vents of the VDVF using the HyBIS TV grab, which also carried a stand-alone pump system to collect particulates. Although these VDVF samples are not undiluted end-member fluids, their ratios of dissolved Fe:Mn, Fe:H 2 S and Mn:H 2 S are at least an order of magnitude lower than those reported for the Rainbow and TAG hydrothermal vent fields on the Mid-Atlantic Ridge ( Table 1 ; elemental ratios are compared with those from TAG and Rainbow as representatives of high-temperature vent fields in mafic and ultramafic settings). These ratios reflect a proportionally high concentration of H 2 S in the emanating fluids at VDVF combined with a low concentration of dissolved Fe relative to Mn. Concentrations of solid-phase Fe, Mn and Cu in particulates from the VDVF are also lower than those at Rainbow and TAG ( Table 1 ). Table 1 Geochemistry of fluids and particles from the Mid-Cayman spreading centre. Full size table The BVF Located at a depth of 4,960 m on the neovolcanic axis of the MCSC, the BVF lies 880 m deeper than the previous deepest known vent field at Ashadze-1 on the Mid-Atlantic Ridge [31] . The BVF consists of a sulphide mound 80 m in diameter and 50 m high ( Fig. 1d ), surmounted with several actively venting sulphide chimneys ( Fig. 4c,d ). An area of weathered sulphide rubble extends for a further 800 m to the east of the active mound. Buoyant vent fluids and particulates collected from an altitude of <5 m above the active chimneys of the BVF differ in geochemical composition to those of other known vent sites. Although these BVF samples are not undiluted end-member fluids, their ratios of Cu:Fe and Cu:Mn in dissolved and particulate phases are at least an order of magnitude higher than those at the Rainbow and TAG hydrothermal vent fields ( Table 1 ). Ratios of Fe:H 2 S and Mn:H 2 S at the BVF are lower than those of other sites, while the ratio of dissolved Fe:Mn shows a similar order of magnitude. The hydrothermal plume from the BVF rises ∼ 1,100 m into the water column, as shown by particulate anomalies measured by LSS ( Fig. 3a ). This contrasts with other vent fields, where buoyant plumes typically only rise 200–400 m into the water column [7] . Using our CTD data and an equation that describes the penetration of a buoyant hydrothermal plume into an overlying water column [32] , we calculate a buoyancy flux ( B o ) of order 10 −1 m 4 s −3 for the BVF hydrothermal plume, which is an order of magnitude greater than that found at other vent sites [33] . Three 'free' parameters might account for such a high buoyancy flux: the exit temperature of the vent fluid, the venting area and the exit vertical velocity. Salinity is not generally considered to have an important role in controlling the magnitude of the buoyancy flux in hydrothermal systems [33] . Using video images of the vent site from the HyBIS vehicle, we estimate the vent area to be of order 0.1–0.2 m 2 , and the exit velocity to be 0.5–1.5 m s −1 . Figure 3c shows the effect of varying exit temperature on plume rise height with these values of vent area and exit velocity. Our analysis therefore indicates that an exit temperature of ∼ 500 °C may be required to achieve the observed plume rise height of 1,100 m above the BVF. Vent fauna of the MCSC The faunal assemblage at the VDVF is dominated by dense aggregations of alvinocaridid shrimp around the actively venting orifices of the edifice peak ( Fig. 4a,b ; greater than 2,000 individuals m −2 ). We observed at least two morphotypes of shrimp at this site, and collected specimens of the numerically dominant type. We recorded zoarcid fish, resembling the genus Pachycara , in video images among the shrimp aggregations at this site, as well as small turrid gastropods and lysianassoid amphipods on fresh sulphide surfaces. We also found solitary galatheid squat lobsters towards the base of the vent edifice. At the BVF, we observed and sampled dense aggregations of the same dominant morphotype of alvinocaridid shrimp as at the VDVF ( Fig. 5a ; greater than 2,000 individuals m −2 ). These shrimp occurred on vent chimneys, and around crevices issuing visible diffuse flow in the central region of the mound, along with high abundances of anemones ( Fig. 5b ; greater than 20 individuals m −2 ) and extensive mats of filamentous microbes on the surfaces of mound sulphides. We encountered occasional macrourid fish in the vent field, and solitary galatheid squat lobsters on the peripheral talus slope of the mound. 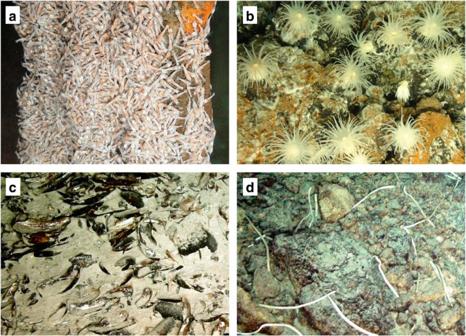Figure 5: MCSC faunal observations. (a) Aggregation of alvinocaridid shrimp on an active chimney at the BVF. (b) Anemones and microbial mats at the BVF. (c) Aggregation of dead mussel shells on the Mount Dent OCC. (d) Empty tubes resembling those of siboglinid polychaetes on the Mount Dent OCC. Figure 5: MCSC faunal observations. ( a ) Aggregation of alvinocaridid shrimp on an active chimney at the BVF. ( b ) Anemones and microbial mats at the BVF. ( c ) Aggregation of dead mussel shells on the Mount Dent OCC. ( d ) Empty tubes resembling those of siboglinid polychaetes on the Mount Dent OCC. Full size image Shrimp specimens collected from both vent fields exhibited similar morphology, with a greatly reduced rostrum, and a four-lobed dorsal organ similar in appearance to the photoreceptor of Rimicaris species [34] . Based on morphology, the MCSC vent shrimp appear to belong to an undescribed alvinocaridid species within the Rimicaris-Chorocaris-Opaepele clade [35] . This relationship is confirmed by the absence of fixed substitutions in partial 16S mitochondrial sequences (549 bp) between the MCSC shrimp and that of Chorocaris chacei , and 0.47% divergence between the partial 16S mitochondrial sequences of MCSC shrimp and Rimicaris exoculata . Although partial 18S nuclear sequences (576 bp) show very few mutations across hydrothermal vent shrimp species, the MCSC shrimp have a fixed substitution in their 18S sequence compared with all other alvinocaridid 18S sequences available in GenBank, and a 0.88% divergence with Rimicaris exoculata . This is consistent with morphological indications that specimens from both MCSC vent fields belong to a single new species. Comparative COI results were inconsistent with morphology and results from 16S and 18S, and may reflect the presence of more than one gene in the COI region. On the upper slopes of the Mount Dent OCC, ∼ 400 m south of the VDVF, we observed an aggregation of mussel shells ( Fig. 5c ) and empty tubes superficially resembling those of siboglinid polychaetes ( Fig. 5d ). No currently active sources of venting or seepage were apparent in the immediate vicinity of this dead assemblage. High-temperature hydrothermal vent fields are known from the neovolcanic axes of all mid-ocean ridges, and in faulted ultramafic settings on slow- and ultraslow-spreading ridges [7] , [36] . Through its occurrence on the upper slopes of an OCC, the VDVF represents a new off-axis setting for high-temperature hydrothermal activity. The presence of anhydrite in mineral samples from the peak of the edifice demonstrates that vent temperatures of at least 140 °C occur at the VDVF, which hosts abundant populations of vent fauna. The VDVF also exhibits sulphide mineralogy in the active part of the mound, and dissolved sulphide in vent fluids. These features therefore contrast with the off-axis Lost City vent field on the Atlantis Massif of the Mid-Atlantic Ridge, where carbonate mineral deposits and cooler (<40–90 °C) sulphide-free fluids are produced by a serpentinization-driven system that hosts a sparse vent fauna [37] . The VDVF is located 13-km west of the axial neovolcanic zone of the MCSC and at an elevation of 2,700 m above it ( Fig. 1b ). In the Nibelungen hydrothermal field at 8°18′S on the Mid-Atlantic Ridge, high-temperature hydrothermal venting occurs 9 km away from the spreading centre axis [38] . Unlike the VDVF, however, the off-axis Nibelungen field occurs in an ultramafic fault-scarp setting, and does not host visible vent fauna [38] . The VDVF therefore represents the furthest off-axis occurrence of high-temperature hydrothermal activity associated with a seafloor spreading centre, and the first active system on an OCC known thus far to support a high abundance of vent fauna. High-temperature hydrothermal activity at Nibelungen field is proposed to be supported by residual heat mined from the deep lithosphere, rather than magmatic processes, via shallow fluid circulation in a non-transform discontinuity [38] . At the Kairei vent field on the Central Indian Ridge, however, high-temperature hydrothermal activity occurs at the top of the rift valley wall, in a similar setting to the VDVF though horizontally and vertically closer to the ridge axis [39] and not associated with an OCC. The high-temperature venting at Kairei is thought to be driven by mining of a heat source at the ridge axis. We propose that high-temperature hydrothermal activity at the VDVF may be similarly supported by deep fissuring on the Mount Dent OCC, allowing the mining of heat from a deep crustal source. The anomalously low ratios of Fe:H 2 S and Mn:H 2 S in fluids at this site ( Table 1 ) may result from the cooling and mixing of ascending fluids in such a pathway, leading to deposition of the metals in an extensive sulphide stockwork and emission of particulate-poor vent fluids. OCCs are common features of slow- and ultraslow-spreading ridges [20] , [21] . Recent studies of several OCCs at 13°N Mid-Atlantic Ridge show ridge-parallel fissuring and intrusion by mafic magmas that are a common and necessary process for the terminal stages of OCC development [40] . Furthermore, extinct hydrothermal sulphide mounds have been found across the upper foot-wall of these Mid-Atlantic Ridge OCCs, indicating that this setting of hydrothermal activity may be more common than hitherto thought [41] . The mechanism supporting high-temperature hydrothermal activity at the VDVF may therefore support active high-temperature vent fields in similar settings at slow- and ultraslow-spreading ridges. However, such off-axis vent fields may be difficult to detect in traditional hydrothermal plume surveys, because of their particulate-poor neutrally buoyant plumes. As global estimates of the incidence of high-temperature vent fields are derived from plume survey data, vent field occurrence may therefore be underestimated along slow- and ultraslow-spreading ridges, which together constitute ∼ 33% of the global mid-ocean ridge system [42] . A greater occurrence of high-temperature hydrothermal vent fields along such ridges also has implications for mineral exploration at mid-ocean ridges [43] and the connectivity of populations of vent fauna [23] . The BVF occurs at a depth ∼ 20% greater than any other known vent site [31] . Although our HyBIS TV grab was not equipped with a manipulator arm and therefore not capable of measuring the temperature of undiluted black smoker fluids directly, we predict exceptionally high-temperature venting at the BVF from two independent lines of evidence. First, the vent fluids collected from <5 m above the chimneys of the BVF are highly enriched in copper, as shown by their high Cu:Fe and Cu:Mn ratios. These ratios are consistent with extremely high-temperature venting at the seafloor [44] and phase separation during hydrothermal circulation, where copper is preferentially enriched in the vapour phase and iron concentrates in the brine phase [45] , [46] . Second, the hydrothermal plume of the BVF rises ∼ 1,100 m above the seafloor, in contrast with other vent fields [8] , where the plume rise height is typically 200–400 m. Our analysis, based on observations of the vent plume in the water column of the MCSC, suggests that a seafloor exit temperature of ∼ 500 °C may be required to produce the observed plume rise height above the BVF. The highest sustained vent fluid temperature known at a deep-sea hydrothermal vent is 407 °C measured in a post-eruptive vent field at a depth of 3,000 m on the Mid-Atlantic Ridge [47] . The BVF corresponds to the seafloor source of the 'Piccard' plume reported previously on the MCSC [11] . It is unclear whether the VDVF is the seafloor source of the previously described 'Europa' plume, which did not exhibit any signals in particulates or Eh [11] . The source of the 'Europa' plume was proposed to be a low-temperature, alkaline-venting system driven by serpentinization [11] , similar to Lost City at the Mid-Atlantic Ridge [37] . Although the MCSC vent fauna may be distinct at species level, their assemblages exhibit higher-level taxonomic affinities with the fauna of vent fields on the Mid-Atlantic Ridge [48] , [49] . The distribution of conspicuous taxa at the BVF also resembles that found at deep Mid-Atlantic vent sites [48] , [49] , [50] , with aggregations of alvinocaridid around high-temperature vent sources, surrounded by an abundant population of anemones in areas of diffuse flow. The water at the bottom of the Cayman Trough is consistent with a modified North Atlantic Deep Water with salinity of 34.988 and temperatures of 3.98 °C ( Fig. 2a ) and relatively high levels of oxygen of around 220 μM. This water may enter the Caribbean via the Windward Passage and flow along the Oriente Fracture Zone [51] . Despite the 4,000-km isolation of the MCSC from the contiguous mid-ocean ridge system, its extant vent fauna show similarities to those of the Mid-Atlantic Ridge, rather than assemblages at the closest known cold seeps, 1,500 km away in the Gulf of Mexico [52] . Bathymetry and water column survey To find and investigate hydrothermal vent fields on the MCSC, we used the shipboard Simrad EM120 multibeam echosounder of the RRS James Cook to map the seafloor spreading centre at a 50-m resolution ( Fig. 1b ). We then deployed a Seabird 911 CTD instrument with LSS and redox (Eh) sensor in three areas, to determine the extent of water column anomalies previously observed in three areas along the MCSC [11] . We deployed the CTD instrument package in 'tow-yo' mode, where the instrument is raised and lowered through a portion of the water column while the ship moves along a survey line, to detect and constrain the extent of hydrothermal plumes dispersing horizontally at their neutrally buoyant depth. Having detected neutrally buoyant hydrothermal plumes, we also undertook vertical profiles with the CTD to detect the buoyant column of hydrothermal discharge above vent sites. Modelling of vent exit temperature from buoyant plume rise height We modelled the buoyant hydrothermal plume above the BVF using the following equation [32] : where z * is the penetration height of the plume, B o is the buoyancy flux (m 4 s −3 ) and N is the buoyancy frequency (s −1 ). In this model, a point source of buoyant fluid is assumed to discharge from a flat seafloor. The plume then rises through a stably stratified background characterized by the buoyancy frequency. We calculated the buoyancy flux [33] as: and the buoyancy frequency [33] as: The variables in these equations were evaluated at the seabed ( z =0) as the point source of the hydrothermal fluid. The background potential temperature ( ), salinity (S̄) and potential density ( ρ ) were calculated from the CTD profile near the vent site ( Fig. 2a ) as averages of these properties over the bottom 100 m of the water column. We calculated a background buoyancy frequency ( N ) of 5.1×10 −4 s −1 for the water column above the BVF, from an average over the bottom 1,000 m of the water column. The thermal expansion coefficient α is 2.13×10 −4 °C −1 , the saline contraction coefficient β is 7.5×10 −4 , g is gravity, A is the area of the vent and W the vertical velocity of the vent fluid. Autonomous underwater vehicle missions In each area where our CTD surveys indicated possible underlying hydrothermal vents, we used the Autosub6000 AUV to constrain and map the seafloor sources of hydrothermal plumes. The Autosub6000 AUV was developed at the National Oceanography Centre, Southampton, and equipped with a CTD, Eh sensor and a Simrad EM2000 multibeam sonar capable of mapping seafloor features to a resolution of ∼ 1 m. TV grab operations We examined the seafloor directly using HyBIS(hydraulic benthic interactive sampler), a manoeuvrable deep-water camera and sampling platform manufactured by Hydro-Lek Ltd in the United Kingdom. Unlike conventional remotely operated vehicles, HyBIS is not equipped with a manipulator arm and its vertical position is controlled by its deployment umbilical. The vehicle is equipped with two thrusters for lateral movement, and carries a high-definition video camera with HMI lights. Guided by live high-definition video imagery from the vehicle, we filtered particulates from the buoyant plumes 5 m above active vents using a stand-alone pump system attached to the vehicle, and sampled buoyant plume fluids using a Niskin bottle. We also used a hydraulic grab and a suction sampler to collect geological and faunal specimens for subsequent mineralogical, morphological and molecular phylogenetic analyses. Geochemical analyses of vent fluids and particulates Although the HyBIS TV grab cannot sample undiluted end-member fluids, we positioned the vehicle <5 m above vent orifices to collect buoyant fluid samples using Niskin bottles. The half-life of dissolved ferrous iron is 2.1 min at 25 °C [53] , and we observed vent fluid exit velocities of 1.5 ms −1 . Therefore, while we cannot compare absolute concentrations of vent fluid constituents with primary end-member fluids from other sites, we can compare elemental ratios. Seawater concentrations of the elements of interest are negligible compared with the levels determined here and are therefore unimportant for the calculation of these ratios. We processed water samples from Niskin bottles carried by HyBIS and the CTD immediately after deployments to determine dissolved methane content. We froze water samples at −20 °C for shore-based analysis of dissolved hydrogen sulphide [54] although oxidation of sulphide may have continued during storage, our sulphide ratio data therefore represent minimum possible values. Dissolved and particulate trace metals ( Table 1 ) were analysed using standard methods [55] . Mineralogical analyses Mineral analyses were made petrologically on samples collected by the HyBIS vehicle by visual identification and verified by XRD analyses. As far as possible, individual mineral samples were picked, dried and crushed and measured on a Philips Analytical wavelength dispersive XRD, and measured qualitatively against mineral standards. Molecular phylogenetic analyses Genomic DNA from shrimp specimens collected from the two MCSC vent fields was extracted using a CTAB extraction procedure [56] . Tissues were digested overnight in 600 μl of a 2% CTAB buffer solution (1.4-M NaCl, 0.2% 2-mercaptoethanol, 20-mM EDTA, 100-mM Tris-HCl pH 8 and 0.1 mg ml −1 proteinase K). DNA was then puried by adding chloroform–isoamyl alcohol (24:1), precipitated together with 1 ml of 100% isopropanol, washed with 70% ethanol and resuspended in 50 μl of sterile H 2 O. For the 16S gene, polymerase chain reaction (PCR) amplifications were performed in 20 μl final volume using 16Sar and16Sbr primers [57] and the following conditions: 1× reaction buffer (200-mM Tris pH 8.8, 500-mM KCl, 0.1% Triton X-100 and 2 mg ml −1 bovine serum albumin), 2.5-mM MgCl 2 , 0.12 mM of each dNTP, 0.38 mM of each primers, 1-U Taq DNA polymerase (Bioline), 2.5 μl of template DNA and sterile H 2 O. Thermal cycling parameters used an initial denaturation at 94 °C for 2 min, followed by 40 cycles at 94 °C for 30 s, 52 °C for 1 min, 72 °C for 2 min and a final 5-min extension cycle. For the 18S gene, PCR amplifications were performed in 20 μl final volume using universal primers [57] and the following conditions: 1× of the same reaction buffer than for the 16S, 2-mM MgCl 2 , 0.2 mM of each dNTP, 0.5 mM of each primers, 1-U Taq DNA polymerase (Bioline), 5 μl of template DNA and sterile H 2 O. Thermal cycling parameters used an initial denaturation at 94 °C for 5 min, followed by 30 cycles at 94 °C for 1 min, 64 °C for 1 min, 72 °C for 2 min 30 s and a final 10-min extension cycle. The GenBank accession numbers for the partial sequences of 16S, COI and 18S regions from the MCSC shrimp are JN850606 , JN850607 and JN850608 , respectively. Sequences of other alvinocaridid shrimp used for comparisons are those available in GenBank. Accession codes: The sequence data have been deposited in the GenBank database under accession codes JN850606 , JN850607 and JN850608 . How to cite this article: Connelly, D. P. et al . Hydrothermal vent fields and chemosynthetic biota on the world's deepest seafloor spreading centre. Nat. Commun. 3:620 doi: 10.1038/ncomms1636 (2012).